Molar tooth carbonates and benthic methane fluxes in Proterozoic oceans Molar tooth structures are ptygmatically folded and microspar-filled structures common in early- and mid-Proterozoic ( ∼ 2,500–750 million years ago, Ma) subtidal successions, but extremely rare in rocks <750 Ma. Here, on the basis of Mg and S isotopes, we show that molar tooth structures may have formed within sediments where microbial sulphate reduction and methanogenesis converged. The convergence was driven by the abundant production of methyl sulphides (dimethyl sulphide and methanethiol) in euxinic or H 2 S-rich seawaters that were widespread in Proterozoic continental margins. In this convergence zone, methyl sulphides served as a non-competitive substrate supporting methane generation and methanethiol inhibited anaerobic oxidation of methane, resulting in the buildup of CH 4 , formation of degassing cracks in sediments and an increase in the benthic methane flux from sediments. Precipitation of crack-filling microspar was driven by methanogenesis-related alkalinity accumulation. Deep ocean ventilation and oxygenation around 750 Ma brought molar tooth structures to an end. Molar tooth carbonates (MTCs), or carbonate rocks containing molar tooth structures (MTSs), occur mostly if not exclusively in successions deposited in subtidal environments before 750 Ma (refs 1 , 2 ). The formation of MTCs requires the generation of cracks within unconsolidated sediments, followed by the rapid infilling of such cracks with early diagenetic calcispar before sediment compaction. The formation of molar tooth (MT) cracks have been variously related to subaqueous syneresis [3] , gas bubble expansion resulting from CH 4 , H 2 S or CO 2 degassing [2] , [4] , [5] , [6] and seismic activities [7] , [8] . The disappearance of MTCs at around 750 Ma has been related to the rise of animals [5] , [7] , [8] , [9] , a drop in calcite saturation of seawater [1] , [2] , [10] or an increase in the concentrations of calcite precipitation inhibitors such as Fe 2+ , Mg 2+ , SO 4 2– or PO 4 (refs 1 , 2 , 3 , 11 ). To illuminate the origin of MTCs, we measured the Mg, S and C isotopic compositions of MTCs from the early Neoproterozoic (1,000–750 Ma) Wanlong Formation in southern Jilin Province of North China ( Supplementary Fig. 1 ). In the Wanlong Formation, MTSs are abundant within the thick-bedded argillaceous lime mudstone that is intercalated with the finely laminated limestone ( Supplementary Note 1 and Supplementary Figs 2 and 3a ). Sedimentological evidence, including the predominance of parallel bedding and the lack of subaerial exposure structures, indicates that MTCs in the Wanlong Formation was deposited below fair-weather wave base [12] . S isotopic data indicate that MT microspar was precipitated within microbial sulphate reduction (MSR) zone and Mg isotopic data suggest that microspar precipitation predated the dolomitization of host rock. We propose that MT microspar was precipitated in the sediment column where MSR and methanogenesis occur simultaneously underneath sulphidic seawaters and where the production of CH 4 from methyl sulphides and the inhibition of CH 4 oxidation by methanethiol allowed CH 4 to build up in the sediments. Petrographic observations of the MTCs MTSs are normally oriented vertically or obliquely with respect to bedding planes and show clear cross-cutting relationships with each other ( Supplementary Fig. 3b–d ). MT cracks are filled with microcrystalline calcite crystals (MT microspars) ranging from 10 to 20 μm in size ( Supplementary Fig. 3e,f ). The argillaceous host rocks (with an average siliciclastic content of 33.4 wt%, Supplementary Table 5 ) are partially dolomitized ( Supplementary Fig. 3g,h ). Isotopic compositions of the MTCs Sulphur isotopic values of carbonate-associated sulphate (CAS) extracted from MT microspars ( δ 34 S MT : 31.9–42.8‰) are higher than those of CAS from calcareous host rock ( δ 34 S HR : 19.1–27.6‰; Fig. 1a , Supplementary Fig. 4 and Supplementary Table 2 ). 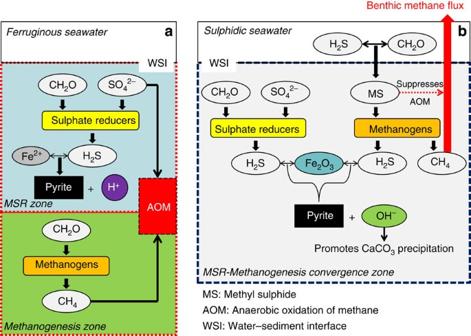Figure 2: Schematic diagram showing geochemical reactions within marine sediments bathed beneath ferruginous and sulphidic seawaters. (a) Under ferruginous conditions, the MSR and methanogenesis zones are separated. Methanogens are outcompeted by sulphate-reducing bacteria, if both use competitive substrates (CH2O)n. Within the MSR zone, reaction between H2S and Fe2+precipitates pyrite and generates H+, which lowers porewater pH. Most CH4produced within methanogenesis zone is oxidized by sulphate at the base of MSR zone where AOM occurs. Thus, there is little benthic CH4flux from marine sediments. (b) Under sulphidic conditions, methyl sulphides are produced within both water column and sediments. In sediments, methyl sulphides serve as a non-competitive substrate for methanogens, allowing MSR and methanogenesis to take place concurrently in the MSR-methanogenesis convergence zone. H2S and Fe2O3react to produce pyrite and generate OH–, thus favouring CaCO3precipitation. AOM is prohibited by methanethiol, allowing CH4accumulation in sediments and significant benthic CH4fluxes into atmosphere. Mg isotopic compositions of MT microspars ( δ 26 Mg MT ) is around –3.3‰ (relative to DSM3), ∼ 1.6‰ lower than those of the host rock ( δ 26 Mg HR ; Fig. 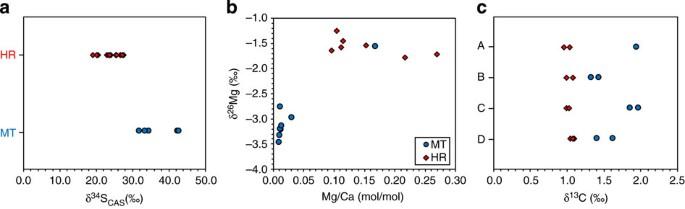1b , Supplementary Fig. Figure 1: Isotopic compositions of MTCs. (a) S isotopic compositions of CAS from MT calcispars (MT) and host rocks (HR). (b) Cross-plot of Mg/Ca (molar ratio) versusδ26Mg. The argillaceous host rock has higher Mg/Ca ratios and is enriched in26Mg than MT calcispars. (c) C isotopic compositions of MT calcispars (MT) versus host rock (HR) of four samples (A, B, C and D). 5 and Supplementary Table 1 ). C isotopes of MT microspars ( δ 13 C MT ) are systematically heavier than host rock ( δ 13 C HR ) by 0.5–1‰ ( Fig. 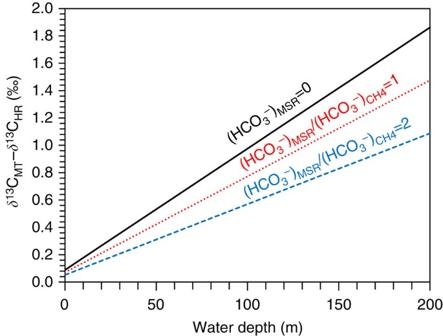Figure 3: Geochemical model showing the carbon isotopic difference between MT microspar and host rock formed at different water depths. First, the amount of CH4required to produce a unit volume of cracks at ambient pressure and temperature was estimated. The co-production ofrelated to CH4generation was then estimated and assumed to have been used fully for MT microspar precipitation. The methanogenicwas inadequate to precipitate enough MT microspar to fill a unit volume and the shortage was made up by (1) pore water(black solid line); (2)from MSR () and methanogenesis () with a molar ratio of 1:1, and the remaining shortage fulfilled by pore water(red dotted line); or (3)from MSR and methanogenesis with a molar ratio of 2:1, and the remaining shortage fulfilled by pore water(blue dashed line). Porewaterwas assumed to have aδ13C value similar to that of host rock (that is, 1‰). Theδ13C value of methanogenicwas estimated at +150‰, given aδ13C value of methyl sulphides at –30‰, a fractionation between CH4and methyl sulphides at –60‰ and the production of 3/4 mole of CH4and 1/4 mole offrom each mole of methyl sulphides (equations (2) and (3)). Theδ13C value of MSRwas assumed to be –30‰. Thexaxis represents water depths and theyaxis indicates the isotopic difference between MT microspar and host rock (δ13CMT-δ13CHR). 1c and Supplementary Table 3 ). Figure 1: Isotopic compositions of MTCs. ( a ) S isotopic compositions of CAS from MT calcispars (MT) and host rocks (HR). ( b ) Cross-plot of Mg/Ca (molar ratio) versus δ 26 Mg. The argillaceous host rock has higher Mg/Ca ratios and is enriched in 26 Mg than MT calcispars. ( c ) C isotopic compositions of MT calcispars (MT) versus host rock (HR) of four samples (A, B, C and D). Full size image δ 34 S HR of the Wanlong carbonates is within the range of sulphur isotopic compositions of Neoproterozoic CAS [13] . The greater values of δ 34 S MT indicate that MT microspar was precipitated in the sulphate reduction zone in the sediment column, where 32 S is preferentially removed from the porewater sulphate pool by sulphate reduction microbes [14] (Supplementary Note 2). MT microspar precipitation in the MSR zone is also consistent with generally lower CAS concentrations in MT microspar than in host rock ( Supplementary Fig. 6 and Supplementary Table 4 ). δ 26 Mg MT is related to the Mg isotopic composition of porewater ( δ 26 Mg pw ), from which MT microspar precipitates, and the relationship can be expressed as follows: where Δ cal is the fractionation associated with inorganic precipitation of low-Mg calcite and can be set at 2.2–2.7‰ (refs 15 , 16 ). Thus, δ 26 Mg pw is estimated to be between –0.6 and –1.1‰, within the range of seawater compositions in the past 70 million years [17] , [18] . Greater δ 26 Mg HR values might be attributed to the partial dolomitization of host rock, because dolostone is systematically heavier than limestone in Mg isotopes [19] , [20] . On the other hand, as dolomite and other authigenic Ca carbonate formed in the sediment column would preferentially scavenge 24 Mg from porewater [21] , [22] (Supplementary Note 3), δ 26 Mg pw would increase as dolomitization proceeds. It is estimated that 10–25 wt% of carbonate in the host rock of the Wanlong Formation is dolomitized ( Fig. 1b ), meaning δ 26 Mg pw would increase by ∼ 2‰ ( Supplementary Fig. 7 ). Had MT microspar in the Wanlong Formation precipitated after host rock dolomitization, seawater Mg isotopic composition would have to be between –2.6 and –3.1‰, which is even lower than the influx from carbonate weathering (–2.25‰; that is, the lower bound of riverine input) [18] . Thus, MT microspar precipitation must predate host rock dolomitization. This inference is also consistent with the petrographic observation that MT structures are often ptygmatically folded and sometimes brittly fractured [1] , suggesting that MT microspar was precipitated before host rock cementation. In this light, it is possible that the exclusive occurrence of MT structures in argillaceous carbonates [1] may be related to clay minerals, which tend to delay host rock cementation [23] . Thus, sedimentary evidence, S isotopes and Mg isotopes indicate that MT microspar precipitation must occur in unconsolidated sediments, within the MSR zone and before dolomitization. To generate MT structures, cracks must develop in unlithified sediments and gas expansion is a plausible mechanism to generate such cracks [2] , [4] . Here we explore the nature of the gases and the unique Proterozoic environments conducive for gas bubble formation in sediments. During the early to middle Proterozoic, atmospheric oxygen level was extremely low (<1% present atmospheric level) and the deep ocean remained anoxic and sulphidic in places [24] , [25] , [26] , [27] . Sulphidic conditions were particularly common in Proterozoic continental margins [25] , [26] , [28] and perhaps in epicratonal environments as well [29] , [30] . Although euxinia may have extended over <10% of global seafloor in mid-Proterozoic according to some estimates [27] , sulphidic waters might have had profound impacts on the Proterozoic Earth system. We propose that methyl sulphides might have been produced in significant quantities in sulphidic marine environments. Methyl sulphides are a group of volatile organic sulphur compounds, including dimethyl sulphide (CH 3 SCH 3 ) and methanethiol (CH 3 SH), which are produced in modern marine and freshwater environments. Methyl sulphides can be produced either by the degradation of dimethylsulphoniopropionate in the surface ocean [31] or by anaerobic methylation of hydrogen sulphide in sulphidic sediments [32] . Therefore, it is expected that the production of methyl sulphides would be enhanced in Proterozoic sulphidic marine environments, both in the water column and within sediments. As volatile gases, methyl sulphides produced in water column tend to readily emit to atmosphere, but those generated within the sediments can serve as a non-competitive substrate for methanogens [33] , [34] , [35] . As sulphur-reducing microbes cannot use methyl sulphides but methanogens can, MSR and methanogenesis can co-occur simultaneously within sediments where methyl sulphides are present [36] , resulting in the convergence of the MSR and methanogenesis zones. In addition, anaerobic oxidation of methane (AOM) is inhibited by methyl sulphides such as methanethiol. With methane oxidation inhibited, CH 4 can accumulate in sediments in significant quantity [37] , in sharp contrast to modern marine sediments, where the MSR zone lies invariably above the methanogenesis zone [38] , with intensive AOM at the base of MSR zone consuming most CH 4 and consequently modern marine CH 4 discharge accounting for only 2% of the global flux [39] ( Fig. 2 ). Figure 2: Schematic diagram showing geochemical reactions within marine sediments bathed beneath ferruginous and sulphidic seawaters. ( a ) Under ferruginous conditions, the MSR and methanogenesis zones are separated. Methanogens are outcompeted by sulphate-reducing bacteria, if both use competitive substrates (CH 2 O) n . Within the MSR zone, reaction between H 2 S and Fe 2+ precipitates pyrite and generates H + , which lowers porewater pH. Most CH 4 produced within methanogenesis zone is oxidized by sulphate at the base of MSR zone where AOM occurs. Thus, there is little benthic CH 4 flux from marine sediments. ( b ) Under sulphidic conditions, methyl sulphides are produced within both water column and sediments. In sediments, methyl sulphides serve as a non-competitive substrate for methanogens, allowing MSR and methanogenesis to take place concurrently in the MSR-methanogenesis convergence zone. H 2 S and Fe 2 O 3 react to produce pyrite and generate OH – , thus favouring CaCO 3 precipitation. AOM is prohibited by methanethiol, allowing CH 4 accumulation in sediments and significant benthic CH 4 fluxes into atmosphere. Full size image We propose that the accumulation of the insoluble gas CH 4 in the convergence zone provided a physical mechanism to generate cracks in unconsolidated sediments [2] , [4] . Furthermore, the geochemistry within the convergence zone where MSR and methanogenesis overlap could have facilitated the precipitation of calcite to fill such cracks. With the generally low concentrations of Fe 2+ in sulphidic porewaters, pyrite formation would involve the reaction between H 2 S and Fe 2 O 3 . In fact, the host rock of MTCs in the Wanlong Formation contains an average of 0.42 wt% of pyrites ( Supplementary Table 5 ). The overall reactions for pyrite formation fueled by MSR and methanogenesis using methanethiol and dimethyl sulphide can be described as follows: These reactions generate OH − and , which elevate pH, increase porewater alkalinity and favour CaCO 3 precipitation [40] , [41] , [42] . In addition, the dearth of calcite inhibitors such as Fe 2+ and SO 4 2– in sulphidic sediments would also promote rapid precipitation of CaCO 3 (ref. 11 ). δ 13 C MT of the Wanlong carbonate is only slightly greater than δ 13 C HR by 0.5–1‰ ( Fig. 1c ), similar to previous studies showing that MT microspar and host carbonate rock have nearly indistinguishable δ 13 C values [5] , [6] , [43] . To assess the extent of carbon isotope variation between MT microspar and host rock, we consider a simple model where methanogenesis produces sufficient CH 4 to produce cracks that are immediately filled with MT microspar. To generate cracks by CH 4 accumulation, gas pressure must be balanced with the hydrostatic pressure, which is dependent on water depth. Our calculation shows that methanogenesis alone does not generate sufficient bicarbonate (and MT microspar) to fill the cracks that would be created at reasonable water depths by the amount of CH 4 it produces. Thus, MT microspar precipitation was probably supplemented by porewater bicarbonate (which would be isotopically similar to seawater bicarbonate and to δ 13 C host ) and bicarbonate derived from sulphate reduction (Supplementary Note 4). To simplify our calculation, we consider the simplest situation in which bicarbonate derived from methanogenesis was entirely used in MT microspar precipitation, with additionally needed alkalinity coming from porewater (that is, a binary mixing model). Assuming that δ 13 C of methyl sulphides and carbon isotope fractionation during methanogenesis are –30‰ and –60‰ (ref. 44 ), respectively, mass balance consideration requires that δ 13 C of derived from methanogenesis be +150‰ based on equations (3) and (4). Our calculation shows that MT microspar precipitation at 100 m water depth would be ∼ 1‰ heavier than host rock (black solid line in Fig. 3 ) and methanogenesis-derived only accounts for <1% of MT microspar precipitation. Smaller isotopic difference between MT microspars and host rock would be expected if MSR-derived is involved (dashed lines in Fig. 3 ). Figure 3: Geochemical model showing the carbon isotopic difference between MT microspar and host rock formed at different water depths. First, the amount of CH 4 required to produce a unit volume of cracks at ambient pressure and temperature was estimated. The co-production of related to CH 4 generation was then estimated and assumed to have been used fully for MT microspar precipitation. The methanogenic was inadequate to precipitate enough MT microspar to fill a unit volume and the shortage was made up by (1) pore water (black solid line); (2) from MSR ( ) and methanogenesis ( ) with a molar ratio of 1:1, and the remaining shortage fulfilled by pore water (red dotted line); or (3) from MSR and methanogenesis with a molar ratio of 2:1, and the remaining shortage fulfilled by pore water (blue dashed line). Porewater was assumed to have a δ 13 C value similar to that of host rock (that is, 1‰). The δ 13 C value of methanogenic was estimated at +150‰, given a δ 13 C value of methyl sulphides at –30‰, a fractionation between CH 4 and methyl sulphides at –60‰ and the production of 3/4 mole of CH 4 and 1/4 mole of from each mole of methyl sulphides (equations (2) and (3)). The δ 13 C value of MSR was assumed to be –30‰. The x axis represents water depths and the y axis indicates the isotopic difference between MT microspar and host rock ( δ 13 C MT - δ 13 C HR ). Full size image The disappearance of MTCs is coincident with the elevation of atmospheric oxygen levels at ∼ 750 Ma (refs 1 , 45 ), suggesting a possible causal relationship. A direct consequence of ocean oxygenation and ventilation is the reduction of the areal coverage of euxinic waters and decrease in methyl sulphide production, which in turn would result in the spatial separation of the MSR and methanogenesis zones in sediments. As such, most CH 4 was consumed at the base of MSR zone by AOM, preventing crack formation by CH 4 accumulation. Furthermore, pyrite formation in ferruginous sediments through reaction with Fe 2+ would generate protons, lowering porewater pH and favouring CaCO 3 dissolution [46] , [47] . All these secular changes associated with atmospheric and oceanic oxygenation may have contributed to the disappearance of MT structure around 750 Ma. CH 4 accumulation in sediments also implies benthic CH 4 discharge from marine sediments. The environmental impacts of benthic CH 4 fluxes on the Proterozoic Earth system could potentially be profound. First, enhanced CH 4 discharge would contribute to the persistently low atmospheric O 2 levels in Proterozoic [25] , [48] . Second, strong benthic CH 4 fluxes from continental margins would have contributed to the maintenance of an ice-free Earth in the middle Proterozoic. Finally, a significant reduction of CH 4 discharge associated with the 750 Ma oxygenation event might have triggered the Neoproterozoic global glaciations. Thus, the Neoproterozoic oxygenation event may have had an impact on the secular distribution of sedimentary structures such as MT structure and the global climate system, as well as the rise of animals [45] . Mg isotope analysis Rock samples were split into two parts using a rock saw. A highly polished slab was prepared from one split, while a mirrored thin section was made from the counterpart. Sample powers were drilled from the polished slab using a hand-held micro-drill. The sampling procedure was guided by the petrographic observation of the corresponding thin sections. For Mg isotopic analysis, about 10–30 mg of powder was dissolved in 0.5 N acetic acid in a 15-ml centrifuge tube. Tubes were placed in an ultrasonic bath for 30 min, to allow complete dissolution of carbonate components. After centrifuging, supernatant was collected for column chemistry and elemental composition analysis. Mg was purified using cation-exchange chromatography. The detailed procedure of column chemistry was reported in Shen, et al. [49] and Huang et al. [20] Mg was purified in two steps. Column 1 was designated to separate Mg from Ca. Mg was eluted by 4 ml of 10 N HCl, whereas Ca was retained in resin. Column 2 was used to separate Mg from all other elements. Na, Al, Fe and K were sequentially eluted using 1 N HCl, 1 N HNO 3 +0.5 N HF and 1 N HNO 3 , whereas Mg was collected using 5 ml of 2 N HNO 3 . To obtain a pure fraction of Mg, sample solutions passed through column 1 twice, followed by three passes through column 2. After column chemistry, Ca/Mg, Na/Mg, Al/Mg and Fe/Mg ratios were <0.05 and the Mg recovery rate was better than 99%. Mg isotopic ratios were measured on a Thermo Scientific Neptune Plus high-resolution multicollector inductively coupled plasma mass spectrometry at the Isotope Laboratory in China University of Geosciences, Beijing. The standard-sample bracketing method was used to correct the instrumental mass bias and drift. An in-house solution (FZT) was used as the working standard. Analyses were performed in the low-resolution mode, simultaneously measuring 26 Mg, 25 Mg and 24 Mg isotopes. Mg isotope ratios are reported by the delta notation as ‰ deviation relative to the DSM3 standard [50] : where x refers to 25 or 26. The internal precision was determined on the basis of ≥3 repeated runs of the same sample solution during a single analytical session and is better than ±0.10‰ (2 s.d.). The accuracy is determined by the measurements of synthetic solution (GSB-Mg) and USGS basalt standards (BCR-2). Multiple analyses of the synthetic solution (GSB-Mg) yield δ 26 Mg values ranging from –2.07 to –2.04‰, which is consistent with the preferred value of –2.05±0.05‰ (2 σ ). δ 26 Mg of BCR-2 is –0.17±0.06‰ (2 σ ), consistent with the published values [51] , [52] , [53] , [54] . Sulphur isotope analysis Traditional CAS extraction procedure typically requires >20 g of carbonate powder. Thus, it is impossible to collect enough sample powder from MT microspar without contamination from the host rock using the traditional method, because MT cracks are typically a few millimetres in width. To analyse CAS of MT microspar, we devised a new extraction procedure that only requires ∼ 1 g of carbonate powders for each sample. The validity of the new procedure was verified by analysing the same carbonate sample by using both the traditional and new procedures. Powders were carefully drilled from MT microspar only to a shallow depth so as to avoid the potential contamination from host rock. Often, multiple MT cracks in a polished slab were drilled to collect enough powder for CAS extraction. Sample powder was placed in a 50-ml centrifuge tube and were treated with 10% NaCl solution for 24 h to dissolve non-CAS sulphate. After supernatant removal, residues were washed with deionized water for three times. The above cleaning procedures were repeated at least three times, to ensure complete removal of non-CAS sulphate. The cleaned sample powder was dissolved in 40 ml of 3 N HCl. After 1 h of reaction, reaction tubes were centrifuged and the supernatants were collected. About 1–2 mg of nano-SiO 2 was added into the centrifuge tube and then 10 ml of saturated BaCl 2 was added to precipitate sulphate as barite. The use of nano-SiO 2 was to facilitate barite collection. Barite precipitation was allowed to proceed for 48 h. After centrifuging, barite precipitate was washed by DI water for three times, to remove residual HCl, and then dried in an oven. Sulphur isotopic compositions were measured at Indiana University on a Finnigan Delta V advantage gas source mass spectrometry fitted with a peripheral Costech elemental analyser for on-line sample combustion. Sulphur isotope compositions are reported as ‰ deviation from V-CDT, δ 34 S=( R sample / R V-CDT −1) × 1,000, where R is the ratio of 34 S/ 32 S. Analytical error is ±0.1‰ (1 σ ) as determined from repeated analyses of samples and laboratory standards. The analytical results were calibrated using the standard NBS-127 (20.3‰) and three internal standards: a silver sulphide (ERE-Ag 2 S: −4.3‰), a chalcopyrite (EMR-CP: +0.9‰) and a barite (PQB2: +40.5‰). Inductively coupled plasma optical emission spectrometer analysis Elemental compositions were determined at Peking University on a Spectro Blue Sop inductively coupled plasma optical emission spectrometer fitted with a Water Cross-flow nebulizer. All analyses were calibrated by a series of gravimetric standards with different concentrations (ranging from 0.1 to 10 p.p.m.) that were run before sample measurements and between every 20 samples. The external reproducibility for the major and minor elements (Na, Mg, Al, K, Ca, Fe, Mn, Sr and S) is ±2%. How to cite this article : Shen, B. et al. Molar tooth carbonates and benthic methane fluxes in Proterozoic oceans. Nat. Commun. 7:10317 doi: 10.1038/ncomms10317 (2016).